Experimental observation of quantum chaos in a beam of light The manner in which unpredictable chaotic dynamics manifests itself in quantum mechanics is a key question in the field of quantum chaos. Indeed, very distinct quantum features can appear due to underlying classical nonlinear dynamics. Here we observe signatures of quantum nonlinear dynamics through the direct measurement of the time-evolved Wigner function of the quantum-kicked harmonic oscillator, implemented in the spatial degrees of freedom of light. Our setup is decoherence-free and we can continuously tune the semiclassical and chaos parameters, so as to explore the transition from regular to essentially chaotic dynamics. Owing to its robustness and versatility, our scheme can be used to experimentally investigate a variety of nonlinear quantum phenomena. As an example, we couple this system to a quantum bit and experimentally investigate the decoherence produced by regular or chaotic dynamics. Chaotic classical systems have the characteristic trait of being extremely sensitive to initial conditions. This behaviour, together with the experimental imprecision of the initial conditions, causes these deterministic systems to be inherently unpredictable. The field of quantum chaos addresses the question as to how classical chaotic dynamics manifests itself in quantum mechanics. In addition to fundamental questions concerning the correspondence principle and the classical limit of quantum mechanics, a number of intriguing quantum-dynamical features have been unravelled. Prominent examples are dynamical localization [1] , [2] , the quantum suppression of classical diffusion and the enhancement of the tunnelling rate in the presence of chaos in the corresponding classical dynamics [3] , [4] . These phenomena have been observed in several physical systems [3] , [4] , [5] , [6] , [7] , [8] , [9] , [10] , [11] , [12] . The simplest and most widely studied systems that present manifestations of classical chaos in their quantum dynamics are periodic time-dependent Hamiltonian (Floquet) systems [13] . The quantum evolution up to discrete time t = nT is described by the quantum map where n is an integer and the Floquet operator U describes the unitary quantum evolution in the time period T . In addition to extensive study from a theoretical viewpoint, the phenomena arising in these maps have been observed in experiments with atoms [2] , [3] , [4] , [5] , [6] , [7] , [8] , [9] , [14] , Bose–Einstein condensates [10] and photonic lattices [12] . There have been a few theoretical proposals to realize quantum chaotic maps using paraxial optics [15] , [16] , [17] and, in fact, dynamical localization has been observed in an optical field sent through a sequence of phase gratings [11] . However, the realization of the quantum-kicked harmonic oscillator (KHO), a paradigm of quantum non-linear dynamics with non-Kolmogorov-Arnold-Moser (non-KAM) behaviour, and a model for charges moving in time-dependent fields [18] , electronic transport in semiconductor lattices [19] , [20] and trapped ions in a periodic laser field [21] , is still outstanding. The quantum KHO is described by the map (1), where the iteration operator is The operator R α describes the evolution of a quantum harmonic oscillator parameterized by α = ωT , where ω is its frequency and T the interval between the periodic perturbations. V K describes a periodic perturbation corresponding to a potential K cos( Q + φ ), where φ is a phase and Q is the dimensionless position variable defined below. The dimensionless position and momentum coordinates of a particle of mass m submitted to the KHO evolution are defined as Q = νq and P = νp /( mω ), respectively, where q and p are the position and momentum of the particle and ν is the spatial frequency of the kick. The dimensionless operators obey [ Q , P ]= iħ eff , where the effective Planck constant is ħ eff ≡ ν 2 ħ / mω . This model can present a rich variety of intriguing quantum-dynamical phenomena [22] , [23] . In the so-called quasicrystal condition and also for irrational values of α , a quantum localization, similar to that extensively studied and observed in the kicked rotor model, can appear [24] . For the crystal condition where α ∈ { π /3, π /2,2 π /3, π ,2 π }, the quantum system can present diffusion in energy for any value of K . In this case, the stroboscopic phase space of the corresponding classical system is characterized by the appearance of a ‘stochastic web’ associated with the chaotic behaviour, with periodic regions corresponding to essentially regular dynamics in between. Stochastic webs are typical structures of systems with non-KAM behaviour, where chaotic dynamics appear even for an arbitrary small perturbation (in our case the kicks) [18] , with have many applications [20] . The size of the web and the perturbation of the regular dynamics inside the periodic regions are governed by the intensity of the perturbation K . For K <1 the size of the web is considerably small, as is the perturbation of the regular dynamics inside the periodic regions. When K =2, the KHO can be considered a weakly chaotic system. Here, we implement the quantum KHO dynamics in the spatial degrees of freedom of the photons of a monochromatic paraxial light. We observe the non-linear dynamics through direct measurement of the optical Wigner function. Controllable parameters adjust the system from regular to chaotic dynamics, as well as the effective Planck constant, associated with the quantum-classical transition. Our scheme is decoherence-free and can be used in a variety of studies of non-linear quantum systems, which we illustrate by investigating the decoherence induced by our system on a qubit. Optical implementation of the chaotic quantum map We implement an optical version of the operator (2) in the spatial degrees of freedom of monochromatic paraxial light based on the isomorphism between the paraxial wave equation and the Schrödinger equation (refs 25 , 26 , 27 and Supplementary Note 1 ). The light beam is sent n times through a combination of optical elements designed to implement the operator U KHO , as illustrated in Fig. 1a . The transverse position in the near and far-field correspond to the position and momentum of the photons in the beam, and are analogous to the transverse position q and transverse momentum p of a quantum particle. 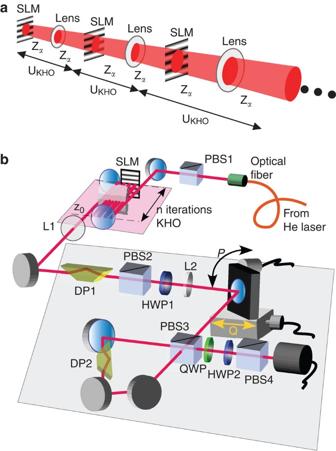Figure 1:Opticalscheme and experimental setup. (a) Illustration of an optical system to implement the quantum KHO. (b) Experimental setup for the implementation of the quantum KHO and measurement of the spatial Wigner function. The output of the He–Ne laser is horizontally polarized using a polarizing beam splitter (PBS1) and reflected intoniterations of the KHO operation. Each iteration consists of a ‘kick’, corresponding to a phase imprinted on the field with the SLM, and harmonic evolution, implemented with sections of free propagation and a cylindrical lens. The beam is reflected back and forthntimes onto the SLM. Lenses L1 and L2 map the final state at transverse planez0onto the entrance of a Sagnac interferometer. Before entering the interferometer, a Dove prism (DP1) is used to perform a 90° spatial rotation of the beam profile, and a polarizing beam splitter (PBS2) and a half-wave plate (HWP1) are used to balance the intensities of the vertical and horizontal polarization components. The interferometer is used for direct measurement of the optical Wigner function. Each phase space point of the Wigner function is obtained from the interference between horizontal (H) and vertical (V) polarization components of the beam emerging from the interferometer. A Dove prism (DP2) inside the interferometer is used to spatially rotate the counter-propagatingHandVcomponents of the field. Translation and tilting of the input mirror are used to select the phase space point (Q,P) to be measured. A quarter-wave plate (QWP), a half-wave plate (HWP2) and a polarizing beam splitter (PBS4) are used to perform the required polarization measurement, and a large aperture power metre is used to measure the beam intensity. See Methods for more information. The instantaneous ‘kick’ perturbation, Figure 1: Optical scheme and experimental setup. ( a ) Illustration of an optical system to implement the quantum KHO. ( b ) Experimental setup for the implementation of the quantum KHO and measurement of the spatial Wigner function. The output of the He–Ne laser is horizontally polarized using a polarizing beam splitter (PBS1) and reflected into n iterations of the KHO operation. Each iteration consists of a ‘kick’, corresponding to a phase imprinted on the field with the SLM, and harmonic evolution, implemented with sections of free propagation and a cylindrical lens. The beam is reflected back and forth n times onto the SLM. Lenses L1 and L2 map the final state at transverse plane z 0 onto the entrance of a Sagnac interferometer. Before entering the interferometer, a Dove prism (DP1) is used to perform a 90° spatial rotation of the beam profile, and a polarizing beam splitter (PBS2) and a half-wave plate (HWP1) are used to balance the intensities of the vertical and horizontal polarization components. The interferometer is used for direct measurement of the optical Wigner function. Each phase space point of the Wigner function is obtained from the interference between horizontal ( H ) and vertical ( V ) polarization components of the beam emerging from the interferometer. A Dove prism (DP2) inside the interferometer is used to spatially rotate the counter-propagating H and V components of the field. Translation and tilting of the input mirror are used to select the phase space point ( Q , P ) to be measured. A quarter-wave plate (QWP), a half-wave plate (HWP2) and a polarizing beam splitter (PBS4) are used to perform the required polarization measurement, and a large aperture power metre is used to measure the beam intensity. See Methods for more information. Full size image is produced using a Holoeye spatial light modulator (SLM). The SLM imprints a programmable phase exp[ i f ( x , y )] on an optical beam, and thus can be used in the implementation of many dynamical maps. We define Q = νq as the dimensionless version of the near-field variable, q ( Supplementary Note 2 ). The parameter ν is the spatial frequency of the cosine function, K is the kick strength, and the effective Planck constant ħ eff will be defined below. The harmonic evolution operator R α produces a phase space rotation that is equivalent to a fractional Fourier transform (FRFT) of order α (ref. 28 ), which can be implemented using a lens of focal length f placed between two sections of free space of distance z α =2 f sin 2 ( α /2). The dimensionless momentum variable is P = νf ′ θ , where θ is the angle of the paraxial ray and f ′≡ f sin α . The dimensionless operators Q and P obey the commutation relation [25] , [26] , where ħ eff = ν 2 f ′/ k is the dimensionless effective Planck constant ( Supplementary Note 2 ). It is straightforward to manipulate all the relevant parameters in the dynamics of the KHO: by changing the order α of the FRFT (harmonic evolution between kicks), the amplitude K of the cosine phase implemented with the SLM and the spatial frequency ν of this phase (effective Planck constant). The experimental setup is illustrated in Fig. 1b . To characterize the chaotic dynamics, we do a point-by-point direct measurement of the optical Wigner function [28] , [29] using an interferometric method [30] . Details of the full experimental setup are given in the Methods section, and in the Discussion section we show how this scheme can be used as a building block to implement long-time dynamics. 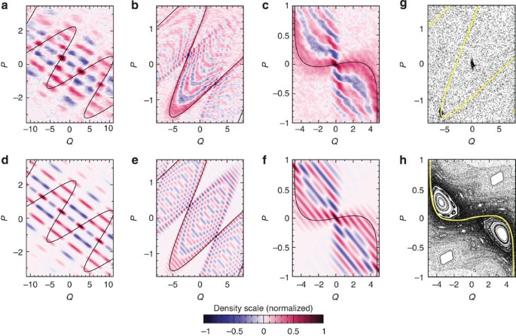Figure 2: Quantum and classical phase space for a single iteration of the KHO map. In the top row from (a) to (c), density plots of the directly measured optical Wigner distributions forn=1 iterations of the KHO map; in the bottom row from (d) to (f), the corresponding numerical predictions. For (a,d), the relevant parameters areK=7.4,ħeff=4.72 andϕ=1.45π; for (b,e),K=7.4,ħeff=0.9 andϕ=1.4π; and for (c,f),K=2,ħeff=0.9 andϕ=0. In all cases the harmonic evolution parameter isα=π/3. The black line outlines the phase space manifold that is the skeleton of both the quantum and the classical distributions corresponding to the KHO Hamiltonian (see details in the text). The associated stroboscopic phase space evolution of the classical map is illustrated in (g,h) corresponding to the cases in (b,c), respectively (the skeleton manifold of the evolved state is the yellow line). The theoretical plots (including the stroboscopic phase space) are obtained from the evolution of the KHO corrected by a linear transformation (equal for all the plots) that take into account the spurious evolution due to technical imperfections and small alignment errors of the optical elements (Methods). Observing quantum signatures of chaos in phase space Figure 2a–c shows three experimental Wigner distributions for a single iteration ( n =1) of the quantum map (2) applied to a squeezed Gaussian state |Ψ(0)〉 centred at the phase space origin (shown in Fig. 3a ). The theoretical Wigner distributions are shown for comparison in Fig. 2d–f . All three cases correspond to the harmonic evolution α = π /3. The classical dynamics of the KHO map (controlled by the kick amplitude K ) are illustrated with the usual stroboscopic kick-to-kick map in Fig. 2g . Figure 2a ) show results for the kick amplitude K =7.4 that corresponds classically to essentially chaotic dynamics ( Fig. 2g ). Figure 2c shows results for K =2 that correspond to a mixed classical dynamics ( Fig. 2h ). Figure 2: Quantum and classical phase space for a single iteration of the KHO map. In the top row from ( a ) to ( c ), density plots of the directly measured optical Wigner distributions for n =1 iterations of the KHO map; in the bottom row from ( d ) to ( f ), the corresponding numerical predictions. For ( a , d ), the relevant parameters are K =7.4, ħ eff =4.72 and ϕ =1.45 π ; for ( b , e ), K =7.4, ħ eff =0.9 and ϕ =1.4 π ; and for ( c , f ), K =2, ħ eff =0.9 and ϕ =0. In all cases the harmonic evolution parameter is α = π /3. The black line outlines the phase space manifold that is the skeleton of both the quantum and the classical distributions corresponding to the KHO Hamiltonian (see details in the text). The associated stroboscopic phase space evolution of the classical map is illustrated in ( g , h ) corresponding to the cases in ( b , c ), respectively (the skeleton manifold of the evolved state is the yellow line). The theoretical plots (including the stroboscopic phase space) are obtained from the evolution of the KHO corrected by a linear transformation (equal for all the plots) that take into account the spurious evolution due to technical imperfections and small alignment errors of the optical elements (Methods). 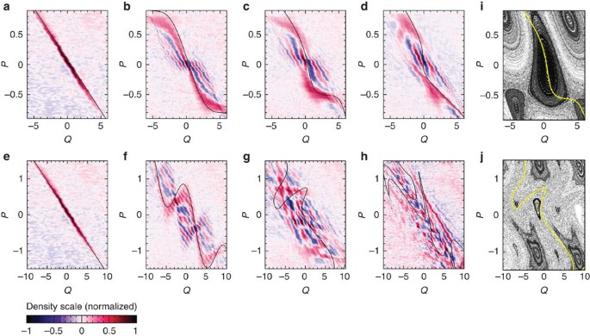Figure 3: Experimentally obtained Wigner distributions corresponding to the first three iterations of the KHO map. The initial Gaussian state is shown in plot (a) (ħeff=0.42) and in (e) (ħeff=0.9). In the top row from (b) to (d), the case of almost regular dynamics, withK=0.75,ħeff=0.42 andϕ=0.44π. In the second row from (f) to (h) the case of weak chaos regime, withK=2,ħeff=0.9 andϕ=1.33π. In all cases,α=2π/3. The corresponding stroboscopic classical phase space are shown in (i) (K=0.75) and (j)K=2. The black lines correspond to the skeleton of both the quantum and the classical distributions corresponding to the KHO (obtained in the same way as inFig. 2). In the bottom row, the recognizable positive skeleton that the Wigner function shares with the classical probability distribution (obtained evolving classically the initial distribution of the Gaussian state) quickly disappear due to the chaotic dynamics (K=2) in comparison with the essentially regular dynamics (K=0.75) pictured in the top row. Full size image Figure 3: Experimentally obtained Wigner distributions corresponding to the first three iterations of the KHO map. The initial Gaussian state is shown in plot ( a ) ( ħ eff =0.42) and in ( e ) ( ħ eff =0.9). In the top row from ( b ) to ( d ), the case of almost regular dynamics, with K =0.75, ħ eff =0.42 and ϕ =0.44 π . In the second row from ( f ) to ( h ) the case of weak chaos regime, with K =2, ħ eff =0.9 and ϕ =1.33 π . In all cases, α =2 π /3. The corresponding stroboscopic classical phase space are shown in ( i ) ( K =0.75) and ( j ) K =2. The black lines correspond to the skeleton of both the quantum and the classical distributions corresponding to the KHO (obtained in the same way as in Fig. 2 ). In the bottom row, the recognizable positive skeleton that the Wigner function shares with the classical probability distribution (obtained evolving classically the initial distribution of the Gaussian state) quickly disappear due to the chaotic dynamics ( K =2) in comparison with the essentially regular dynamics ( K =0.75) pictured in the top row. Full size image Extended quantum states (with uncertainty Δ Q Δ P >> ħ eff /2) typically exhibit a fine oscillatory structure in their Wigner function, known as sub-Planck structure [31] , which saturate at a scale ∼ ħ . Thus, for an almost fixed extension in phase space, the wavelength of the oscillatory pattern should decrease with ħ eff . This can be observed comparing Fig. 2a , where ħ eff =4.72, with Fig. 2b where ħ eff =0.9 (in both cases K =7.4). The Wigner function of some extended states, like energy eigenstates in integrable systems, have a classical manifold as their support. Every pair of localized regions of the Wigner function on this support can interfere creating an oscillatory pattern in the middle of a chord that joins the localized regions, similar to the Wigner function of a superposition of two coherent states (a Schrodinger cat-like state). When the classical dynamics is sufficiently non-linear, the evolution of even highly localized Gaussian states are supported by a phase space manifold that evolves classically [32] , [33] . This is also the skeleton of the classical probability distribution associated with the initial Gaussian state whose evolution is determined by the Liouville equation of the classical system. In all the plots of Fig. 2 , a curve (yellow in Fig. 2g , black in the rest) indicates the classical manifold that is the support of the Wigner function. For our initial squeezed Gaussian state this is a straight line, as in Fig. 3a . The interference pattern appears once the stretching and folding of the classical manifold begins due to the non-linear classical dynamics. Eventually, some portion of the interference pattern falls over the classical support, and the positive skeleton begins to disappear. This occurs very quickly when the underlying dynamics is chaotic. This can be seen in Fig. 3 , which shows the Wigner function of the first three iterations of the KHO map (2) for the same initial state |Ψ(0)〉 (shown in (a) and (e)), when K =0.75 in (b) to (d) and when K =2 in (f) to (h). The non-linear regular classical dynamics of a stability island around the origin for K =0.75 is shown in the stroboscopic phase space plot (i), and the weak chaotic dynamics for K =2 in plot (j). The quantum KHO as a decohering environment As an example of the utility and versatility of our approach, we measured the loss of coherence in a polarization qubit coupled to the quantum KHO, which acts as a decohering environment. By taking advantage of the fact that the SLM only imprints a phase on the horizontal polarization component, a polarization-dependent evolution, KHO or simple harmonic oscillator (SHO), is implemented in the spatial degrees of freedom (Methods). This corresponds to a dephasing-type interaction between qubit and environment. In this case, the off-diagonal elements of the qubit density matrix are suppressed by a factor , where |Ψ(0)〉 is the initial state of the environment. Thus, for an initial state of the qubit in the equatorial plane of the Bloch sphere, the temporal behaviour of its purity is given by (1+| f | 2 )/2. The quantity f can be seen as a fidelity amplitude, which has been extensively studied in the field of quantum chaos [34] , [35] , [36] . In general, theoretical studies predict an initial decay of f before saturation [34] , [35] , [36] . For fully chaotic underlying classical dynamics, f presents an exponential decay with different decay rates depending on the perturbation regime [34] , [35] . On the other hand, for regular dynamics, the decay of f is not generic and depends strongly on the localization of the initial state in the classical phase space [34] , [35] . For initial states well localized in a stability island long time oscillations with revivals are expected, where the oscillations can be understood in terms of the classical frequencies included in |Ψ(0)〉. The temporal mean value of f decreases with ħ eff so, due to revivals, the size of the fluctuations increase in the semiclassical regime. When the underlying dynamics of the environment is chaotic the temporal mean value of f and its fluctuations are inversely proportional to the effective Hilbert space dimension of the environment [36] and therefore tend to 0 in the semiclassical limit ( ħ eff →0). In this limit the qubit becomes maximally entangled to the environment, so its purity→1/2. In our experiment, an incoming beam was prepared in a linear diagonal polarization state. 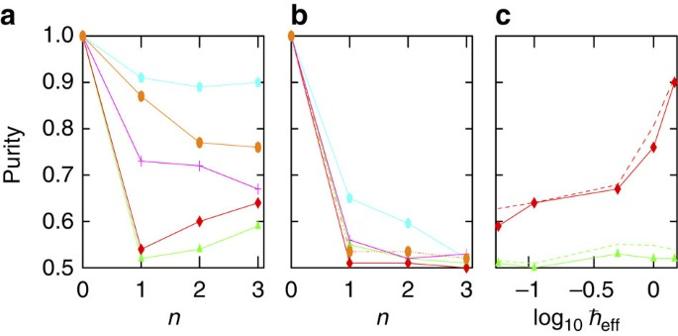Figure 4: Purity loss of the diagonal polarization state for regular and chaotic dynamics of the environment. Purity as a function of the number of KHO iterations,n, for (a) regular dynamics (K=0.5) and (b) chaotic dynamics (K=2). In both figures,α=2π/3 andħeff=0.05 (green triangles), 0.1 (red diamonds), 0.5 (purple crosses), 1.0 (orange circles) and 1.5 (blue polygons). (c) The final purity as a function ofħeffforn=3 KHO iterations, withK=2 (green triangles) andK=0.5 (red diamonds). The dashed lines show the predictions given by numerical simulation of the composite qubit-KHO system. The solid lines joinling the experimental points are only to assist visualization. Figure 4a show the purity of the polarization state as a function of the number of iterations of the KHO map. Figure 4a is for essentially regular dynamics ( K =0.5), and Fig. 4b shows the case in which the KHO has chaotic dynamics ( K =2). The initial state |Ψ(0)〉 is analogous to the one shown in Fig. 3a and in the case when K =0.5 is localized in an stability island around the origin (not shown). Figure 4c shows the purity for n =3 kicks as a function of ħ eff for K =2 (green triangles) and K =0.5 (red diamonds). The dashed lines are the predictions given by numerical simulation of the composite system. Although the number of kicks are few, one observes a general behaviour compatible with the theory described above. In the case of chaotic dynamics ( K =2), rapid loss of purity occurs for all values of ħ eff attaining a saturation with very small fluctuations, indicating that the polarization state becomes nearly maximally entangled (purity=1/2) for decreasing values of ħ eff ( Fig. 4c ). Hence, the equilibrium state of the qubit is a totally mixed state. The total loss of coherence in the polarization state here is due to the underlying classical chaotic dynamics in the spatial degrees of freedom of the beam. On the other hand, for regular dynamics ( K =0.5), because |Ψ(0)〉 is almost completely localized in an stability island, we observe what appears to be the beginning of oscillations for different values of ħ eff , with a revival of the polarization state purity (for all values of ħ eff ). The value of the purity at its minimum value goes to 1/2 in the semiclassical limit ( Fig. 4c ), indicating that the temporal mean value of f goes to 0 when ħ eff →0. This is compatible with the typical large fluctuations of the fidelity amplitude f in the semiclassical regime for the case of regular dynamics when the initial state is localized in a stability island. Figure 4: Purity loss of the diagonal polarization state for regular and chaotic dynamics of the environment. Purity as a function of the number of KHO iterations, n , for ( a ) regular dynamics ( K =0.5) and ( b ) chaotic dynamics ( K =2). In both figures, α =2 π /3 and ħ eff =0.05 (green triangles), 0.1 (red diamonds), 0.5 (purple crosses), 1.0 (orange circles) and 1.5 (blue polygons). ( c ) The final purity as a function of ħ eff for n =3 KHO iterations, with K =2 (green triangles) and K =0.5 (red diamonds). The dashed lines show the predictions given by numerical simulation of the composite qubit-KHO system. The solid lines joinling the experimental points are only to assist visualization. Full size image The optical KHO setup reported here can be used as a building block to implement a large number of iterations of the KHO operator. 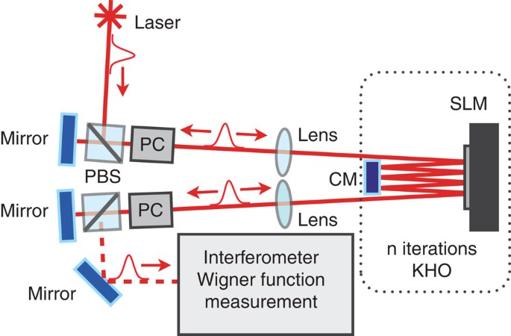Figure 5: Scaling up to a large number of kicks. Theniterations of the KHO operator can be used as a building block forn>>1 kicks. An optical pulse is switched into the setup using a PC. ThenKHO iterations are performed using a cylinder mirror and SLM. After a number of KHO evolutions, the pulse can be switched out of the setup and into the interferometer for direct measurement of the Wigner function.The ultimate limit to the number of iterations that can be performed depends on the losses in the optical system (Supplementary Discussion). Figure 5 shows an experimental scheme that can be used to implement N >>1 kicks of the KHO. A pulse from a vertically polarized laser is reflected from a polarizing beam splitter (PBS), and the polarization is rotated to the horizontal direction by a Pockels cell (PC). The laser is sent to the SLM, and n iterations of the KHO operator are implemented, in the same manner as reported in the Results section. To minimize losses from multiple optical components, a single cylindrical mirror can be used in the place of the cylindrical lens and plane mirror in Fig. 1 . After n iterations, the output light is sent through a second PC, which can be used to switch the pulse out of the setup for measurement. The measurement system is the interferometer used for direct measurement of the spatial Wigner function. If the PC is left inactive, the pulse is reflected from the mirror and backwards through the KHO operation, resulting in another n iterations. The lenses are chosen with focal length equal to half the distance between the SLM and mirrors, so that two consecutive optical Fourier transforms are performed. The overall result is an imaging system, up to a reflection. In this way, the output state from each set of n iterations is mapped onto the input state for the next set of n iterations. As the kick operator (3) and harmonic evolution (4) are symmetric around the origin, the reflections can be absorbed into the definition of the coordinate system. The pulse is sent back to the first PC, which remains inactive, resulting in reflection of the pulse at the mirror, and transmission back into the n KHO iterations. In this way, it is possible to implement a sequence of n × 2 n × 2 n kicks and switch the output state into the interferometer for measurement after the first n iterations, or at intervals of 2 n after that. We note that the SLM allows us to control the number of kicks n per iteration by programming whether the kick phase or a quadratic phase is imprinted on the field. The quadratic phase can be used to implement or undo the harmonic evolution. Figure 5: Scaling up to a large number of kicks. The n iterations of the KHO operator can be used as a building block for n >>1 kicks. An optical pulse is switched into the setup using a PC. The n KHO iterations are performed using a cylinder mirror and SLM. After a number of KHO evolutions, the pulse can be switched out of the setup and into the interferometer for direct measurement of the Wigner function.The ultimate limit to the number of iterations that can be performed depends on the losses in the optical system ( Supplementary Discussion ). Full size image The ultimate limit to the number of iterations that can be performed depends primarily on the losses in the optical system. These arise predominantly from the SLM, lenses and mirrors used in the n iterations of the KHO. The total output intensity after n kicks of the KHO can be written as follows: where t o is the combined transmission coefficient of the optical elements outside the KHO evolution, t l is the combined transmission coefficient of the lenses and mirrors that implement the harmonic evolution between kicks, t SLM the transmission coefficient of the SLM and I in the input intensity of the laser beam. In the Supplementary Discussion , we estimate that with current technology it should be possible to perform about n ∼ 100 kicks. In conclusion, our experiment allows for the study of the dynamics of a non-relativistic quantum system using an intense classical laser beam due to the analogy between quantum mechanics and classical wave mechanics. A possible next step is to study the chaotic evolution of entangled photons. The optical realization of non-linear quantum dynamics should prove invaluable in the experimental investigation of quantum chaos, decoherence and the quantum-classical boundary. Experimental setup The complete experimental setup is illustrated in Fig. 1b . A 632.8-nm He–Ne laser is coupled to a single-mode optical fibre. This defines a Gaussian light beam as the initial state , which is then evolved by the quantum KHO propagator (2) in one dimension of the transverse spatial degrees of freedom. The state is sent through n iterations of the KHO operator U KHO by reflecting n times between the SLM and a mirror. A polarizing beam splitter (PBS1) is used to polarize the beam parallel to the active axis of the SLM display. The harmonic evolution between kicks corresponds to propagation in the α -order fast Fourier transform system, which consists of free space propagation and the cylindrical lens. For practical reasons, we actually implement two consecutive fast Fourier transforms of order α /2, before each incidence on the SLM. The focal length of the cylindrical lens is f =150 mm, and the free space propagation length is z =75mm, so that α = π /3 between two consecutive kicks ( Fig.1b ). As the entire KHO evolution is made with optical elements that act only in one spatial dimension, the perpendicular direction evolves according to free space propagation (see the Supplementary Discussion for details and a discussion of the accessibility of long-time dynamics). To measure the Wigner function, two spherical lenses (L1 and L2) of focal length f =350 mm are used to map the output state of the KHO system | ψ ( n )〉 from the transverse plane at position z 0 to the input mirror of the Sagnac interferometer. A Dove prism (DP1) tilted at a 45° angle is used to swap the horizontal and vertical coordinates, because for convenience the quantum-kicked Hamiltonian is implemented in the vertical axis, whereas the Wigner measurement is performed in the horizontal. The second PBS (PBS2) and the first half-wave plate 1 are used to keep the beam linearly polarized before entering the Sagnac interferometer. Measurement of the optical Wigner function The method used to directly measure the optical Wigner function is an interferometric scheme proposed in (ref. 30 ). The interferometer is illustrated in Fig. 1 . The displacement and tilting of a steering mirror (M1) at the entrance of a three-mirror Sagnac interferometer displaces the optical field by Q and changes its direction of propagation by P (which in the paraxial approximation corresponds to the addition of a phase). This produces the field . A polarizing beam splitter divides the field into two spatially identical components and a Dove prism (DP2) placed inside the interferometer realizes opposite 90° spatial rotations in the two counter-propagating transverse spatial modes, resulting in a total relative rotation by 180°. The modes are recombined, and projected onto the diagonal polarization direction before detection by an area-integrating ‘bucket’ detector. The measured intensity is composed of three terms I = I 1 + I 2 + I int , where the sum I 1 + I 2 is constant and equals half the total input intensity. The term I int originates from the interference between the counter-propagating beams. Owing to the relative rotation implemented by DP2, I int is proportional to: The right-hand side of equation (7) is an integral over spatial variable ξ of the overlap between the displaced field, , and its complex conjugate with the transformation ξ →− ξ . This transformation corresponds to the 180° relative rotation implemented by DP2. It is important to note that slight polarization transformations introduced by the DP [37] inside the Sagnac interferometer does not alter (at all) the measured Wigner function. In this way, the amplitude of the optical Wigner function at point ( Q , P ) can be obtained by measuring the intensity at the interferometer output for different settings of the tilt angle and displacement of the steering mirror M1. In our experiment, these parameters were controlled with high-resolution motorized stages. At the exit of the interferometer we use a quarter-wave plate that is tilted to adjust the relative optical phase between the two arms of the interferometer [37] . Analysis of the experimental data The final state of the optical KHO is obtained at the output plane z 0 , indicated in Fig. 1b . However, the optical wave function propagates through free space and several linear optical elements before reaching the steering mirror at the entrance of the Sagnac interferometer, where the optical Wigner function is measured. One must therefore take into account this evolution before comparing measurements with the theoretical Wigner functions, obtained from numerical calculation of the quantum KHO evolution. This is done by calculating the total linear transformation , resulting from propagation through all of the optical elements and free space between the output plane z 0 and the steering mirror shown in Fig. 1b . The expected Wigner function in the measurement plane can be written as follows: where are the transformed coordinates. The function represents the Wigner function due to KHO evolution of the initial Gaussian state implemented in the x transverse spatial direction. The function refers to the Gaussian state describing the y transverse spatial direction at plane z 0 . This spatial mode does not undergo KHO evolution. Experimental errors associated with the propagation though the optical elements between the output plane z 0 and the steering mirror results in scaling, skewing and rotation of the final measured Wigner function, W (exp) ( x , p x ), in comparison with W (KHO) ( x , p x ). These uncertainties are due principally to errors in lens placement, misalignment of the optical elements and diffraction. Nevertheless, a single linear transformation corrects these errors, such that . Both and depend only on the experimental setup, and are the same for all measurements of Wigner functions, including the case in which the SLM is turned off. In this case, the implemented evolution is that of a SHO. With the KHO turned off, we determined the value of , and used these values to correct all of the KHO Wigner functions. This was repeated for each harmonic evolution used. Implemention of a dephasing-type decoherence channel The SLM imprints a phase on the horizontal polarization component of the light beam, but leaves the phase of the vertical polarization component unchanged. Without the SLM, the optical system is designed to implement SHO evolution via the FRFT systems composed of the cylindrical lens and free space propagation. Therefore, if diagonally polarized light is used in the KHO optical setup, one obtains the transformation: where , and |Ψ〉 designates the transverse spatial mode of the light beam. The evolution operators U KHO and U SHO act on the spatial degree of freedom, and correspond to the evolution of the KHO and the SHO, respectively. The total evolution given in equation (9) could be interpreted as the quantum evolution of a qubit interacting (instantaneously at the moment of each kick) with a quantum KHO via a dephasing type of coupling of the form , where we denote with s H and s V the linear polarization eigenvalues of | H 〉 and | V 〉, respectively, and s = s H or s = s V . Performing a polarization measurement of the output beam using a ‘bucket’ detector is equivalent to tracing over the spatial degree of freedom, and yields, where is the overlap between the SHO and KHO quantum states. The purity of the polarization state is given by Tr ρ 2 =(1+| f | 2 )/2, and decays with f ( [36] ). We use wave plates and a PBS to perform quantum polarization state tomography using the standard recipe [38] , [39] to obtain the density matrix ρ , from which we calculate the results shown in Fig. 4 . How to cite this article : Lemos G. B. et al . Experimental observation of quantum chaos in a beam of light. Nat. Commun. 3:1211 doi: 10.1038/ncomms2214 (2012).